SET activation of nitroarenes by 2-azaallyl anions as a straightforward access to 2,5-dihydro-1,2,4-oxadiazoles The use of nitroarenes as amino sources in synthesis is challenging. Herein is reported an unusual, straightforward, and transition metal-free method for the net [3 + 2]-cycloaddition reaction of 2-azaallyl anions with nitroarenes. The products of this reaction are diverse 2,5-dihydro-1,2,4-oxadiazoles (>40 examples, up to 95% yield). This method does not require an external reductant to reduce nitroarenes, nor does it employ nitrosoarenes, which are often used in N–O cycloadditions. Instead, it is proposed that the 2-azaallyl anions, which behave as super electron donors (SEDs), deliver an electron to the nitroarene to generate a nitroarene radical anion. A downstream 2-azaallyl radical coupling with a newly formed nitrosoarene is followed by ring closure to afford the observed products. This proposed reaction pathway is supported by computational studies and experimental evidence. Overall, this method uses readily available materials, is green, and exhibits a broad scope. Heterocyclic compounds are of great importance in the pharmaceutical and pesticide industries. Among heterocycles, oxadiazoles, five-membered ring heterocycles containing an oxygen and two nitrogens, and their derivatives, have attracted considerable interests [1] , [2] , [3] , [4] , [5] , [6] , [7] , [8] , [9] , [10] . Among oxadiazoles, those containing the 1,2,4-oxadiazole skeleton, including 2,5-dihydro-1,2,4-oxadiazoles, are of interest because of their prevalence in various biologically active compounds (Fig. 1 ). They have been found to exhibit antiviral [11] , anticancer [12] , [13] , anti-inflammatory [14] , antirhinovirus [15] , and antiparasitic properties [16] , [17] , [18] , [19] . They are also known as muscarinic agonists [20] , [21] , [22] , GABA modulators [23] , and benzodiazepine receptor agonists [24] . Fig. 1 Some biologically important compounds containing 1,2,4-oxadiazole core. Full size image Due to the utility of 1,2,4-oxadiazoles in the pharmaceutical industry, their synthesis has received significant attention. Traditional methods for the synthesis of 1,2,4-oxadiazoles are largely based on two approaches (Fig. 2a ): (1) 1,3-dipolar cycloaddition of nitriles to nitrile oxides and (2) thermally promoted cyclization of amidoxime derivatives [25] , [26] . Despite the popularity of these methods, they suffer from limited precursor availability. Recently, Xuan, Xiao, and co-workers developed a [3 + 2]-cycloaddition of 2H-azirines with nitrosoarenes under photoredox catalysis with visible light. In their study, a series of 2,5-dihydro-1,2,4-oxadiazole derivatives were prepared in moderate yields (up to 63%, Fig. 2b ) [27] . A drawback of this, and related cycloadditions [28] , [29] , is the use of nitrosoarenes, which have very limited commercial availability and stability. Fig. 2: Synthetic methods for 1,2,4-oxadiazoles and 2,5-dihydro-1,2,4-oxadiazoles. a Traditional route oxadiazoles. b Cycloaddition under photoredox catalysis. c This work with key intermediates. Full size image In contrast to nitrosoarenes, nitroarenes are feedstocks and represent one of the most readily available starting materials in organic synthesis. They are easily prepared from the parent arenes via Friedel–Crafts nitration and many are commercially available and inexpensive. Recent years have witnessed the use of nitroarenes as amino sources, often in transition metal catalyzed processes [30] , [31] , [32] , [33] , [34] , [35] , [36] , [37] . A more formidable challenge is the use of nitroarenes as amino precursors in the absence of transition metal catalysts [38] , [39] , [40] , [41] , [42] , [43] , [44] , [45] . Herein, we report a transition-metal-free net [3 + 2]-cycloaddition of nitroarenes with 2-azaallyl anions under basic conditions to afford 2,5-dihydro-1,2,4-oxadiazoles in good to excellent yields (Fig. 2c ). A unique reaction mechanism is proposed, wherein single electron transfer (SET) from the 2-azaallyl anion to the nitroarene eventually leads to a 2-azaallyl radical that couples with a newly formed nitrosoarene. Considering the significant role of nitroarenes in various aspects of modern chemistry, we envision that this straightforward method will be of interest in organic synthesis and medicinal chemistry. Background We have been interested in the fascinating chemistry of N -benzyl ketimines, which undergo deprotonation to give 2-azaallyl anions that exhibit umpolung reactivity [46] . In our initial investigations, we studied the use of 2-azaally anions and related pronucleophiles in palladium catalyzed cross-coupling reactions with aryl halides [47] , [48] . In these reactions, the 2-azaally anions were produced in situ from either aldimines or ketimines under basic reaction conditions. Subsequently, we found that 2-azaallyl anions behave as super electron donors (SEDs) [49] , as defined by Murphy and co-workers, and we characterized their reducing properties and the structures of the 2-azaallyl anions and radical [50] . The 2-azaallyl anions promote transition metal-free arylation with aryl iodides and alkylation with sterically encumbered alkyl iodides (Fig. 3a ) [51] , [52] , [53] , [54] . They are synthetically useful for the synthesis of benzofurylethylamines (Fig. 3b ) and their isochromene analogs [55] , [56] . In the presence of bulky aryl iodides, where the coupling in Fig. 3a is slow, cross-dehydrogenative coupling reactions take place. As shown in Fig. 3c , the aryl radical undergoes hydrogen atom transfer (HAT) with ethers (such as tetrahydrofuran (THF), shown), amines, or toluenes. Radical–radical coupling then leads to functionalized products [57] . Fig. 3: SET reactions with 2-azaallyl anions. a Transition-metal-free cross-coupling reactions. b Cyclization/radical-radical coupling processes for the synthesis of benzofurans. c Dehydrogenative cross-coupling reactions. Full size image Reaction development and optimization In the present study, we were interested in capitalizing on the SED properties of 2-azaallyl anions and explored their reactivity with nitroarenes. We initiated our studies with nitrobenzene ( 1a ) and N -benzylidene-1,1-diphenylmethanamine ( 2a ), which leads to a 2-azaallyl anion upon deprotonation. 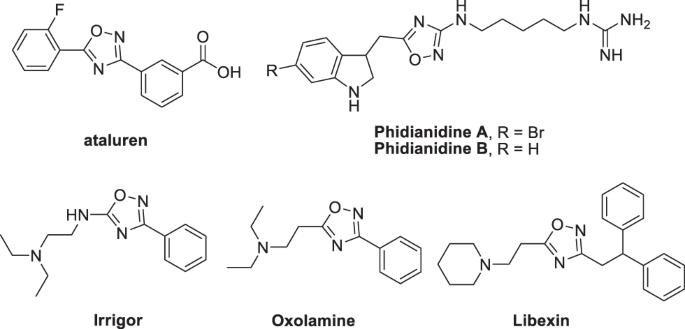Fig. 1 Some biologically important compounds containing 1,2,4-oxadiazole core. For the deprotonation, seven bases were screened in THF [KO t Bu, NaO t Bu, LiO t Bu, LDA, KOH, NaOH, and LiOH] at 100 °C for 12 h (Table 1 , entries 1–7). LDA and KOH caused decomposition of the aldimine and all reactions that did not generate product resulted in recovered nitroarene. Only NaOH and LiO t Bu were suitable bases for the desired transformation, giving the corresponding product 3aa in 35% and 53% yields (entries 2 and 7), respectively. Testing a collection of solvents [1,4-dioxane, DME (dimethoxy ethane), toluene, and CPME (cyclopentyl methyl ether), Table 1 , entries 8–11] indicated that the reaction in THF outperformed those in other solvents. Performing the reaction at 120 °C did not improve the yield (Table 1 , entry 12), while only trace product was observed when the reaction was conducted at 80 °C. The excess amount of aldimine is essential for high conversion (Table 1 , entries 14–17). The yield was elevated to 77% with two equiv. of imine 2a , and 86% yield was obtained when the ratio of imine 2a to nitrobenzene was 3:1. We note that the reaction at RT under blue light gave only 13% yield of the oxadiazole product after 24 h irradiation (entry 18). The structure of 3aa was confirmed by X-ray diffraction (CCDC 2032323). Table 1 Reaction optimization a . Full size table Scope of the aldimine With the optimized reaction conditions in hand (Table 1 , entry 15), the scope of the N -benzyl group of the aldimine partner was examined. As shown in Fig. 4 , various aldimines bearing substituents on the N -benzyl group gave the desired products in moderate-to-good yields (58–95%). Aldimines possessing alkyl groups (4-Me and 3,4-Me 2 ) gave products 3ab and 3ac in 87 and 92% yield, respectively. Substrates bearing electronegative groups and electron-withdrawing substituents (4-Cl, 4-F, 3-CF 3 , and 3-OCF 3 ) underwent reaction in 76–85% yield to furnish the oxadiazole products ( 3ad , 3ae , 3af , and 3ag ). Electron-donating substrates (4-NMe 2 , 4-OPh, 4-OMe, 4-SMe, and 2-OMe) provided desired products ( 3ah , 3ai , 3aj , 3ak , and 3al ) in 61–95% yield. Aldimines possessing biphenyl ( 3am ), 4-pyrazolylphenyl ( 3an ), 4-morpholinophenyl ( 3ao ) and 2-naphthyl ( 3ap ) groups were all tolerated in this protocol, furnishing the cycloaddition products in 75–81% yield. Additionally, aldimines containing heterocycles were also well tolerated. For example, 2-azaallyls bearing 2-furanyl, 3-furanyl, 2-thiofuranyl, and 3-thiofuranyl heteroarenes participated in this reaction, giving the products 3aq – 3av in 58–82% yield. Replacing one of the phenyl groups of 2a with a methyl group to give 2a’ , the oxadiazole product ( 3aa' ) was prepared in 58% yield with NaO t Bu as base. To illustrate the scalability of this method, we conducted the reaction of nitrobenzene ( 1a ) with N -benzhydryl-1-(thiophen-3-yl)methanimine ( 2v ) on a 5 mmol scale. The cyclized product 3av was isolated in 75% yield (1.43 g). Fig. 4: Substrate scope a,b . a Scope of the aldimine. b Scope of the nitroarene. a Reaction conditions: nitroarene (0.1 mmol), aldimine (0.3 mmol), LiO t Bu (0.36 mmol), THF (0.1 M), 100 °C, 12 h. b Isolated yield. c 0.2 mmol of aldimine. d 0.24 mmol of LiO t Bu. e Reaction performed on 5 mmol scale. f 0.36 mmol of NaO t Bu. g DME (0.1 M). Full size image Scope of the nitroarene coupling partner The range of nitroarene substrates was next explored. Nitroarenes bearing diverse substituents exhibited good to excellent reactivity, including those with alkyl (3-Me, 3ba , 85% yield), electron-donating (4-OMe, 3ca , 85% yield), and electronegative or electron-withdrawing substituents [4-OCF 3 ( 3da ), 3-OCF 3 ( 3ea ), 4-Br ( 3fa ), 3-Br ( 3ga ), 4-Cl ( 3ha ), 3-Cl ( 3ia ), 4-CF 3 ( 3ja ), 3-CF 3 ( 3ka ), and 3-F ( 3la ), 71–91% yield]. Nitroarenes possessing 4-Ph ( 3ma ), heterocyclic 2-furanyl and 2-thiofuranyl ( 3na , 3oa ), and benzyl ( 3pa ) groups all worked well in this transformation (77–88% yield). In addition to monosubstituted nitroarenes, disubstituted nitroarenes such as 1-bromo-3-methoxy-5-nitrobenzene 1q , 2-fluoro-1-methoxy-4-nitrobenzene 1r , and 1-methoxy-2-methyl-4-nitrobenzene 1s were also suitable substrates in this protocol, affording the cyclized products 3qa – 3sa in 81–85% yields. These substrates are primed for further functionalization through cross-coupling strategies. Overall, a variety of 2,5-dihydro-1,2,4-oxadiazoles were readily prepared by net [3 + 2] cycloaddition of simple nitroarenes with aldimines. In an effort to broaden the types of oxadiazoles accessible with this method, we targeted 1,3-diaryl 2-azaallyl anions with the goal of preparing triaryl-substituted oxadiazoles. As shown in Fig. 5 , N -benzylidene-1-phenylmethanamine ( 2A ) underwent reaction at 60 °C to afford 3aA in 81% yield. We next wished to examine unsymmetrical 1,3-diaryl 2-azaallyl precursors to explore regioselectivity in this reaction. When the aldimine 2B , prepared from 2-methyl benzaldehyde, was employed, the 2-tolyl group of the product was preferentially located in the sterically least hindered position with a regioisomeric ratio (rr) of 78: 22. The rr of all products was determined by 1 H nuclear magnetic resonance (NMR) analysis of the crude reaction mixture. In the case of 3aB , the major regioisomer was isolated by column chromatography in 70% and its assignment as the 5-tolyl derivative made based on heteronuclear multiple quantum coherence and heteronuclear multiple bond coherence experiments. In contrast, when aldimines 2C – E , generated from 4-halo-benzaldehydes, were employed (halogen = F, Cl, Br) the opposite regioisomer was observed with rr = 35: 65 (X = F), 24: 76 (X = Cl) and 32: 68 (X = Br). The isolated yields of the major regioisomers were 61% ( 3aC ), 55% ( 3aD ), and 50% ( 3aE ). The regiochemistry of the major regioisomer 3aE was further confirmed through characterization by X-ray crystallography (CCDC 2068961). Fig. 5: Substrate scope in the synthesis of triaryl-substituted oxadiazoles and ring-opening products a,b . a Reaction conditions: nitroarene (0.1 mmol), 2a (0.3 mmol), LiO t Bu (0.36 mmol), THF (0.1 M), 60 °C, 12 h. b Isolated yield. c 100 °C. Full size image A brief study of nitroarenes with the 1,3-diphenyl aldimine 2A was performed. Nitroarenes bearing electron-donating (4-OMe), electronegative (4-Br, 4-Cl, 4-F) and electron-withdrawing (4-CF 3 ) substituents were well tolerated in this reaction and furnished the products in 76–90% yield. Furthermore, we were pleased to find that the diversity of the compounds accessible could be extended by increasing the reaction temperature by 40 °C. Thus, when the reaction between 1a and 2A was conducted at 100 °C the N–O bond in the oxadiazole was cleaved and the ring-opening product 3AA was isolated in 88% yield. A succinct study of the cyclization/ring opening reaction was performed with representative nitroarenes bearing electron-donating (4-OMe, 3CA and 4-NMe 2 , 3TA ) and electronegative (4-F, 3LA ) groups. These substrates performed well in this cyclization/ring-opening transformation, giving the products in 69–86% yield. These examples highlight the utility of nitroarenes as amino sources in this chemistry. Interestingly, reaction of 2a’ with nitrobenzene in the presence of LiO t Bu (3 equiv.) at 100 °C resulted in the formation of the ring-opened product 3AA , which has undergone demethylation. Initially, we suspected that 3aa’ from Fig. 4 is formed as an intermediate and underwent demethylation by LiO t Bu. However, subjecting 3aa’ to the reaction conditions gave no 3AA (Fig. 6a ). Thus, demethylation occurs earlier in the reaction. Further, we also conducted the reaction without the addition of PhNO 2 , but the demethylation product was not observed in the recovered materials, which indicated that the demethylation did not occur before the participation of the nitroarene. Fig. 6: Ring-opening experiments. a Demethylation experiment. b Role of base in ring-opening of oxadiazoles. Full size image We were interested in gaining insight into the nature of the ring-opening reactions in Fig. 5 . Thus, subjecting the oxadiazole 3aA to heating at 100 °C in THF for 12 h resulted in recovery of the oxadiazole. When the same reaction was performed in the presence of 2 equiv. LiO- t -Bu, which is necessary for the formation of the oxadiazole, the ring-opened product was obtained in 80% yield. This result suggests that the ring-opening is promoted by base, as shown in Fig. 6b . It is noteworthy that the N -benzoylbenzamidinate products formed in this tandem reaction are useful ligands in the area of materials science, especially for ring opening polymerization processes [58] , [59] , [60] . Mechanistic experiments To probe the mechanism of this unusual transformation, several experiments were conducted. When the nitroarene was subjected to 1 equiv. LiO t Bu for 12 h at 100 °C in THF in the absence of imine, the nitroarene was recovered in 87% yield. This result indicates that the LiO t Bu does not act as the reducing agent to reduce the nitroarene. A competition experiment between 0.1 mmol of 3-fluoro nitrobenzene ( 1l ) and 0.1 mmol 4-trifluoromethyl nitrobenzene ( 1j ) with 0.1 mmol imine 2a in the presence of 2 equiv. LiO t Bu resulted in the formation of product derived from the 4-trifluoromethyl nitrobenzene in 65% yield and no detectable amount of product formed from the 3-fluoro nitrobenzene (Fig. 7a ). The faster reaction of the 4-trifluoromethyl nitrobenzene is consistent with a mechanism involving initial reduction of the nitroarene. Fig. 7: Competition experiments and dimerization of the 2-azaallyl radical. a Competition between two nitroarenes. b Competing reaction pathways between arylation and oxadiazole formation. c Formation of the oxadiazole and diastereomeric dimers through 2-azaallyl radical coupling processes. Full size image Next, we focused on the chemoselectivity between two reactive functional groups. 3-Iodo nitrobenzene 4 has two reactive functional groups that are susceptible to reduction, providing two possible reaction pathways (Fig. 7b ). A reasonable first step in both reactions is SET from the 2-azaallyl anion to 3-iodo nitrobenzene to generate the arene radical anion. The top pathway in Fig. 7b involves loss of iodide from the arene radical anion and generation of an aryl radical. Reaction of the persistent 2-azaallyl radical with the aryl radical would give the tetraaryl product, as was previously reported for aryl iodides not bearing nitro groups (Fig. 3a ) [61] . However, the arylated product was not detected by 1 H NMR spectroscopy under these conditions. Instead, it appears that the reduced nitro arene leads to the oxadiazole product 5 in 64% yield (Fig. 7b , bottom pathway). This reaction is proposed to proceed through nitrosobenzene, as discussed further below. The results of Fig. 7b highlight the lower barrier to reaction at the nitro center vs. loss of iodide. Finally, we note that the dimerization of the 2-azaallyl radical takes place to generate the diimine products, as is commonly observed in reactions of 2-azaallyl anions that proceed through open-shell intermediates (Fig. 7c ). Note that the assay yields (AY) were determined by 1 H NMR integration of the crude reaction mixture. The AY of the diimines are based on the 0.3 mmol aldimine employed in this reaction, whereas the oxadiazole AY is based on the nitrobenzene. Mechanistic studies by DFT Computational studies were carried out to shed light on the mechanistic pathway. First, the deprotonation of aldimine 2a in the presence of LiO t Bu was considered. Two possible adducts between LiO t Bu and the aldimine were examined ( INT1 and INT1ʹ , Fig. 8a ). In INT1 the ketimine 2a binds to LiO t Bu via Li–N dative interaction and in INT1ʹ a cation–π interaction is formed. Computational results show that the cation–π interaction in INT1ʹ is ca. 6 kcal/mol higher in energy than the dative adduct in INT1 . A transition state for deprotonation via the cation–π adduct was located as shown in TS1 , in which the C 3 •••H distance is lengthened to 1.44 Å while O•••H distance is shortened to 1.25 Å. The resulting cation–π complex formed after deprotonation ( INT2ʹ ) is reminiscent of crystallographically characterized structures of 2-azaallyl anions with main group metals [50] . This structure is predicted to rearrange to the more stable adduct INT2 with a Li–N dative interaction. Fig. 8: Computational studies. a Energy profile for the formation of the key 2-azaallyl radical ( 2a′ ) and nitrosobenzene. b Energy profile for the formation of the final product ( 3aa ). Bond distances are shown in Å. Full size image Next, a ligand exchange step between t BuOH and nitrobenzene ( 1a ) generates the O-bound κ 2 -nitrobenzene adduct INT3 . While this step is uphill by 6.4 kcal/mol, INT3 can undergo an exergonic intersphere SET to afford a diradical complex INT3a in triplet state. The open-shell singlet of INT3a was also considered, which was 0.2 kcal/mol higher in energy than the triplet state of INT3a . The SET from the 2-azaallyl anion to the nitrobenzene is downhill by 14.3 kcal/mol. Intermediate INT3a possesses the bound 2-azaallyl radical ( 2aʹ ) and the nitrobenzene radical anion. In addition, substituent effects on the nitroarene were also considered for the SET step. When nitroarene 1j , possessing a 4-CF 3 substituent, and 1l , bearing a 3-F substituent, were used in the calculations, the calculated energy gap for 1j (21.6 kcal/mol) was significantly larger than that of 1l (18.0 kcal/mol), implying that the generation of the corresponding radicals is more efficient for 1j than for 1l . This computational prediction is consistent with the experimental observations that the 4-trifluoromethyl nitrobenzene reacts faster than 3-fluoro nitrobenzene in the competitive experiment shown in Fig. 7a ). We initially expected that diradical intermediate INT3a might undergo internal C–N or C–O bond formation (Supplementary Fig. 1 ). Calculated barriers for these processes, however, exceeded 50 kcal/mol. Thus, we envisioned exchange of the bound 2-azaallyl radical for the aldimine starting material. The liberated 2-azaallyl radical is known to undergo dimerization to afford diimines, which are observed products (Fig. 7c ). The calculations indicate that the lithium salt of the nitrobenzene radical anion, INT4 , can bind to the aldimine 2a through the nitrogen atom to generate a new adduct, INT5 . With the nitrobenzene radical anion and the aldimine 2a both bound to Li + , HAT from the benzylic C–H of the bound aldimine by the oxygen of the nitrobenzene radical anion via TS2 generates INT6 . Hydroxide migrates from the nitrogen of INT6 to lithium to form a complex of the 2-azaallyl radical, nitrosobenzene, and LiOH ( INT7 ) in the coordination sphere of the Li + (Attempts to locate the transition state of hydroxyl migration failed. The favorable electrostatic attractive interaction between Li cation and hydroxyl group is mainly responsible for the facile formation of LiOH from INT6 to INT6’ . ). 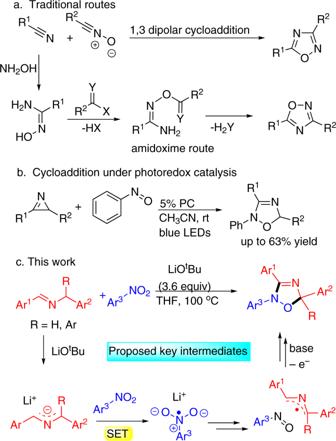Fig. 2: Synthetic methods for 1,2,4-oxadiazoles and 2,5-dihydro-1,2,4-oxadiazoles. aTraditional route oxadiazoles.bCycloaddition under photoredox catalysis.cThis work with key intermediates. Thus, the reduction of PhNO 2 to PhNO is proposed, along with the formation of LiOH. Dissociation of the nitrosobenzene and 2-azaallyl radical is next proposed. After the formation of nitrosobenzene, radical additions with the 2-azaallyl radical 2aʹ were examined computationally. To form the product 3aa , both O-attack of PhNO on C 3 of 2aʹ and N-attack to C 1 were considered (Fig. 8b ). Computational results show that it is more favorable for N-attack at C 1 via TS3b to afford INT9b . One may propose that the subsequent intramolecular O-attack of INT9b at C 3 via TS4b might occur to furnish a cyclized intermediate INT10 . However, computational results show that this cyclization step needs to overcome a much higher activation barrier (41.7 kcal/mol), suggesting that this pathway is not feasible (Supplementary Fig. 2 ). On the other hand, the formed INT9b might undergo a proton transfer step with LiO t Bu via TS4 to afford the radical anion INT11 . Subsequently, the intramolecular cyclization of INT11 could follow via TS5 to afford radical anion INT12 . The calculated activation energy for this step is 31.9 kcal/mol, which is reasonable under these reaction conditions. We also examined the pathway with O-attack of PhNO at C 3 of the 2-azaallyl radical 2aʹ (via TS3a) as the first step in the cyclization, followed by N-attack to C 1 via TS4a to generate the cyclized species. However, the predicted overall activation energy for this pathway is 37.6 kcal/mol (Supplementary Fig. 2 ), which is substantially higher than the proposed pathway shown in Fig. 8b . Finally, the formed radical anion INT12 could undergo SET with nitrobenzene to form the oxadiazole and INT13 . The formed INT13 could undergo another ligand exchange step with substrate 2a to generate the final product 3aa and INT5 , which enters a next cycle. Mechanistic considerations Grounded in the computational and experimental results above, and observations reported in the literature, a reaction mechanism is provided in Fig. 9 and discussed here. Deprotonation of the aldimine 2 generates the 2-azaallyl anion. Given that reactions with stronger bases, such as LDA, do not give the oxadiazole products in appreciable yields, we interpret these observations to suggest that low concentrations of the 2-azaallyl anion, or downstream intermediates like the 2-azaallyl radical, are crucial to the success of this reaction. The strong base LDA would rapidly convert the aldimine to the 2-azaallyl anion, depleting the aldimine, which is a key intermediate as seen in Fig. 8b . As noted above, SET from the 2-azaallyl anion to the nitroarene is proposed to afford the nitroarene radical anion, A . It is noteworthy that the radical anion of nitrobenzene has been characterized experimentally and computationally [62] , [63] . As might be expected, most of the increased electron density on forming the nitrobenzene radical anion is located on the nitro group [63] . From electrochemical data it is known that the reduction of nitroarenes occurs more readily than the reduction of aryl iodides [64] . Nonetheless, as shown in Fig. 3a , in the absence of a nitro group, 2-azaallyl anions reduce aryl iodides to aryl radicals [51] , [52] , [53] , [54] . Also formed in this SET step is the persistent 2-azaallyl radical, which undergoes dimerization to form the rac - and meso -diimines outlined in Fig. 7c . Fig. 9: Proposed reaction pathway. Key steps include reduction of the nitroarene by the 2-azaallyl anion, HAT from the aldimine to the nitroarene radical anion ( B ), formation of the nitrosoarene ( D ), and radical-chain propagation from G . Full size image Based on the computational study, the nitroarene radical anion A does not react with the 2-azaallyl radical. Instead, calculations show a lower barrier for HAT between the lithium bound nitro arene radical anion and the aldimine via the arrow pushing shown in B . The next step involves elimination of LiOH via C . The products of this step are a nitrosoarenes and the 2-azaallyl radical. We then set out to determine whether the nitrosoarene was a viable intermediate in this reaction, as shown in Fig. 10 . In the presence of 4-nitrotoluene and 4-nitroso anisole, imine, and base, the net [3 + 2] product was formed from the nitrosoarene, consistent with the calculations. The 2-azaallyl radical and nitrosoarene undergo addition to form the C–N bond in E with a lower barrier than the formation of the C–O bond (Fig. 8b ). Intermediate E is proposed to undergo deprotonation by LiO t Bu and isomerization via F to afford the radical anion ( G ). 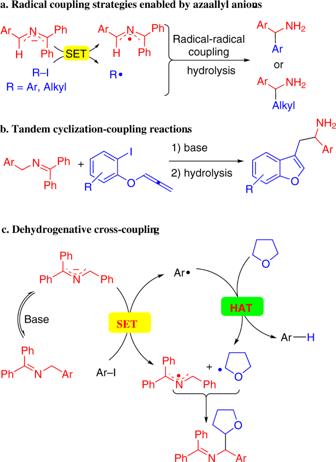Fig. 3: SET reactions with 2-azaallyl anions. aTransition-metal-free cross-coupling reactions.bCyclization/radical-radical coupling processes for the synthesis of benzofurans.cDehydrogenative cross-coupling reactions. Radical chain propagation occurs when G transfers an electron to a nitroarene to regenerate the nitroarene radical anion and the oxadiazole product 3 . Fig. 10: Competition reaction with nitrosoarene. Product 3ca is consistent with the intermediacy of the nitrosoarene in the net [3+2] reaction. Similar results were obtained with 4-nitro anisole and 4-nitrosotoluene, which gave 3ta (not shown). Full size image We have developed a transition-metal-free reaction of aldimines with nitroarenes. This method provides a green and operationally simple approach to afford a variety of 2,5-dihydro-1,2,4-oxadiazole derivatives in good yields. The scope of the reaction is broad with high functional group compatibility and enables rapid incorporation of heteroaryl groups. 2,5-Dihydro-1,2,4-oxadiazoles belong to a class of biologically important heterocyclic compounds that are employed in the pharmaceutical industry and found in natural products. This new protocol is distinct from previously reported cycloadditions, because it involves nitroarenes rather than nitrosoarenes. 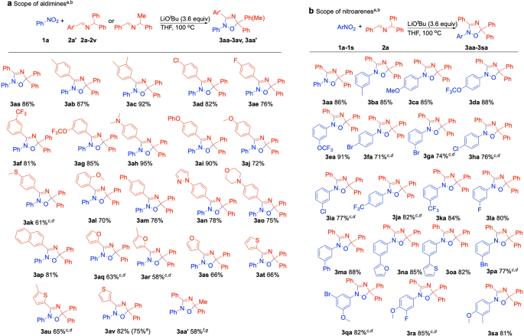Fig. 4: Substrate scopea,b. aScope of the aldimine.bScope of the nitroarene.aReaction conditions: nitroarene (0.1 mmol), aldimine (0.3 mmol), LiOtBu (0.36 mmol), THF (0.1 M), 100 °C, 12 h.bIsolated yield.c0.2 mmol of aldimine.d0.24 mmol of LiOtBu.eReaction performed on 5 mmol scale.f0.36 mmol of NaOtBu.gDME (0.1 M). Nitroarenes are abundant, commercially available feedstocks, but have proven difficult to employ as amino sources in organic synthesis. A unique aspect of this reaction is the distinct mechanism, where the 2-azaallyl anion serves to activate the nitroarene by SET, eliminating the need for external reducing agents. Computational studies suggest that the lowest energy pathway involves a radical-chain process. Considering the great potential of nitroarenes in the chemical sciences, we envision that this new protocol will be of interest in modern chemistry and hope that it inspires chemists to revisit the use of nitroarenes as amino sources. 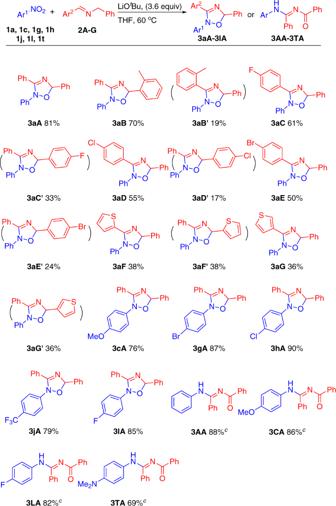Fig. 5: Substrate scope in the synthesis of triaryl-substituted oxadiazoles and ring-opening productsa,b. aReaction conditions: nitroarene (0.1 mmol),2a(0.3 mmol), LiOtBu (0.36 mmol), THF (0.1 M), 60 °C, 12 h.bIsolated yield.c100 °C. General procedures for synthesis of 3aa An oven-dried 10 mL vial equipped with a stir bar was charged with aldimine (0.3 mmol) and LiO t Bu (28.8 mg, 0.36 mmol) under a nitrogen atmosphere in a glovebox. THF (1 mL) was added to the reaction followed by addition of nitroarene (10.2 μL, 0.1 mmol) by syringe at room temperature. The color of the reaction mixture turned to light yellow. The vial was capped, removed from the glovebox, and stirred for 12 h at 100 °C. After cooling to room temperature, the reaction mixture was quenched with three drops of H 2 O, and the vial was open to air, passed through a short pad of silica gel, and eluted with ethyl acetate (1 mL × 3). 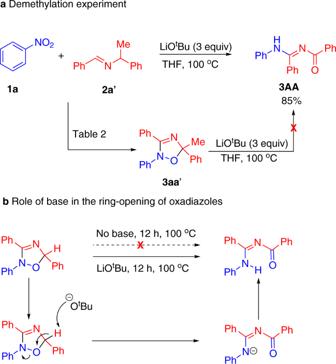Fig. 6: Ring-opening experiments. aDemethylation experiment.bRole of base in ring-opening of oxadiazoles. The combined organic solution was concentrated under reduced pressure. 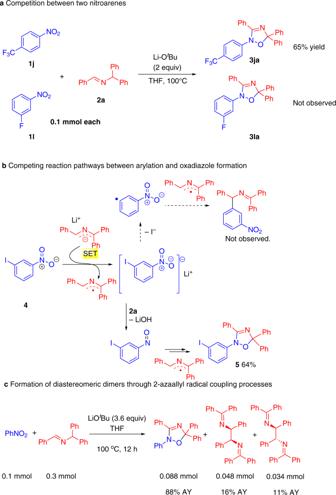Fig. 7: Competition experiments and dimerization of the 2-azaallyl radical. aCompetition between two nitroarenes.bCompeting reaction pathways between arylation and oxadiazole formation.cFormation of the oxadiazole and diastereomeric dimers through 2-azaallyl radical coupling processes. 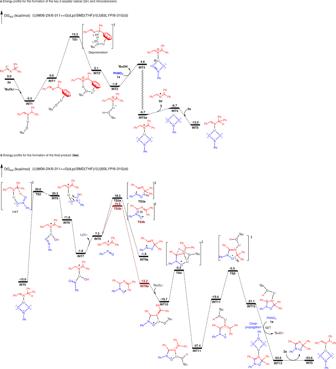Fig. 8: Computational studies. aEnergy profile for the formation of the key 2-azaallyl radical (2a′) and nitrosobenzene.bEnergy profile for the formation of the final product (3aa). Bond distances are shown in Å. 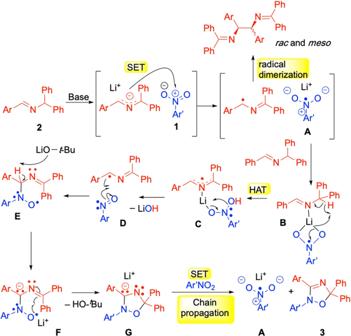Fig. 9: Proposed reaction pathway. Key steps include reduction of the nitroarene by the 2-azaallyl anion, HAT from the aldimine to the nitroarene radical anion (B), formation of the nitrosoarene (D), and radical-chain propagation fromG. 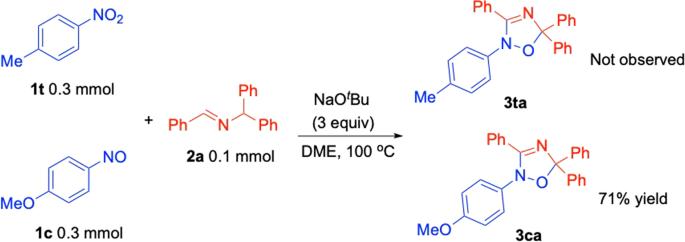Fig. 10: Competition reaction with nitrosoarene. Product3cais consistent with the intermediacy of the nitrosoarene in the net [3+2] reaction. Similar results were obtained with 4-nitro anisole and 4-nitrosotoluene, which gave3ta(not shown). The crude material was loaded onto a silica gel column and purified by flash chromatography.